Lsr2 acts as a cyclic di-GMP receptor that promotes keto-mycolic acid synthesis and biofilm formation in mycobacteria 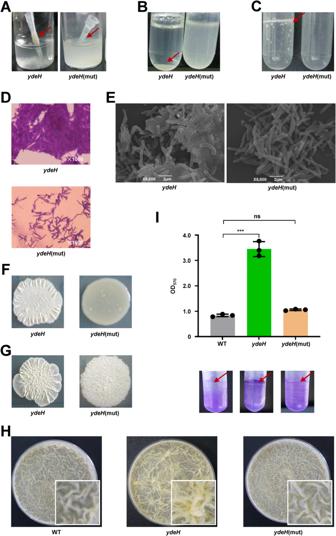Fig. 1: c-di-GMP controls biofilm formation byM. smegmatis. AAdhesion of theydeH, andydeH(mut) strains.BSedimentation rate of theydeH(mut), andydeHstrains.CPellice formation of theydeH, andydeH(mut) strains.DThe cells morphology of theydeH, andydeH(mut) strains after staining with 2% crystal violet under light microscope.EScanning electron microscopy assays of cell morphology forydeH, andydeH(mut) strains. The images were taken at 8000x magnification. The experiments of (D–E) were performed three times and the representative images were shown.FColonial morphology of theydeHandydeH(mut) strains on LB agar plates.GColonial morphology of theydeHandydeH(mut) strains on 7H10 agar plates.HBiofilm formation at the air–liquid surface of the wild type,ydeHandydeH(mut) strains.IQuantitation of biofilm biomass by crystal violet staining of the wild type,ydeHandydeH(mut) strains (n= 3, biological replicates). Two-tailed t-tests were performed for statistical analysis (***p= 0.0001). Data were presented as mean ± SD. The source data were provided in the Source data file. Cyclic di-GMP (c-di-GMP) is a second messenger that promotes biofilm formation in several bacterial species, but the mechanisms are often unclear. Here, we report that c-di-GMP promotes biofilm formation in mycobacteria in a manner dependent on the nucleoid-associated protein Lsr2. We show that c-di-GMP specifically binds to Lsr2 at a ratio of 1:1. Lsr2 upregulates the expression of HadD, a (3R)-hydroxyacyl-ACP dehydratase, thus promoting the synthesis of keto-mycolic acid and biofilm formation. Thus, Lsr2 acts as a c-di-GMP receptor that links the second messenger’s function to lipid synthesis and biofilm formation in mycobacteria. Cyclic di-GMP (c-di-GMP), a conserved second messenger in bacteria, regulates several important physiological processes, including biofilm formation [1] , motility [2] , and virulence [3] . Generally, under high levels of intracellular c-di-GMP, bacteria tend to grow in biofilms rather than as a planktonic cells [4] . Recently, it has been reported that c-di-GMP promotes biofilm formation mediated by elongation factor P in Acinetobacter baumannii [5] . c-di-GMP also interacts with its effector BpfD to regulate biofilm formation in Shewanella putrefaciens [6] . However, the regulatory mechanism by which c-di-GMP regulates biofilm formation and the receptor involved in mycobacteria remain unknown. Biofilms are a critical structured community for bacterial adaptation to harsh environmental conditions. Several mycobacterial species, including Mycobacterium tuberculosis , have been shown to form biofilms in vitro [7] , [8] . Mycobacteria have a lipid bilayer cell wall structure in which lipid components account for 60% (wt/wt) of the cell wall weight [9] . A variety of lipids have been reported to play important roles in mycobacterial biofilm formation [10] , [11] , [12] . The extracellular matrix of mycobacterial biofilms is rich in mycolic acid, an important lipid component of the cell wall [13] , [14] . Moreover, an increased c-di-GMP concentration has been shown to increase the production of keto-mycolic acid (keto-MA) in Mycobacterium bovis BCG [15] . However, the signal regulatory pathway by which c-di-GMP regulates keto-MA synthesis is still unclear. Lsr2 is a nucleoid‑associated protein (NAP) responsible for maintaining a highly organized chromosome structure and transcriptional regulation in mycobacteria, including M. smegmatis [16] and M. tuberculosis [17] , [18] . As a global regulator, Lsr2 regulates biofilm formation [19] , [20] , [21] , [22] and the cell cycle [23] in M. smegmatis . In M. tuberculosis , Lsr2 extensively regulates antibiotic resistance [24] , oxidative stress [25] , and virulence [18] . Mutation of Lsr2 led to smooth colony generation and deficient biofilm formation in M. smegmatis [19] , [21] . However, the regulatory pathway by which Lsr2 regulates biofilm formation remains largely obscure, especially in terms of upstream regulatory signals and downstream target genes. HadD is a (3R)-hydroxyacyl-ACP dehydratase of the fatty acid synthase type II (FAS-II) system. It has been reported that HadD is involved in FAS-II elongation cycles during the synthesis of MA in mycobacteria [26] , [27] . hadD deletion alters the composition of MA and its relative lipids, leading to impaired rough colony generation and biofilm formation [26] . However, the upstream regulatory pathway of HadD in mycobacteria is still unclear. Here, we found that Lsr2 is a receptor for c-di-GMP, with a binding ratio of 1:1. Lsr2 plays a crucial role in c-di-GMP by regulating colony morphology and biofilm formation in mycobacteria. In addition, Lsr2 positively regulated biofilm formation by triggering the expression of HadD to synthesize keto-MA, a lipid of the mycobacterial cell wall. Moreover, our study demonstrates that c-di-GMP stimulates Lsr2 activity to positively regulate the expression of hadD . Therefore, our study revealed the signaling pathway through which the c-di-GMP combines with the receptor Lsr2 to control biofilm formation. This finding reveals the links among second messenger, lipids, and mycobacterial biofilm formation. High levels of c-di-GMP affect colony morphology and biofilm formation of M. smegmatis In our preliminary experiments, we found that overexpression of the diguanylate cyclase (DGC) gene ydeH from Escherichia coli in M. smegmatis resulted in bacterial adhesion to pipette tips. To explore the molecular mechanism underlying this strange phenomenon, we constructed a high c-di-GMP-content M. smegmatis strain by overexpressing ydeH ( ydeH ) and a control strain ( ydeH (mut)) by overexpressing the mutant ydeH gene [28] . Surprisingly, high levels of c-di-GMP significantly altered the bacterial phenotypes, including increasing adhesion (Fig. 1A ), sedimentation (Fig. 1B ), and pellicle at the air–liquid surface (Fig. 1C ). Furthermore, under a light microscope, the accumulation of ydeH resulted in robust crystal violet staining (Fig. 1D ). A similar result was found by scanning electron microscopy, as ydeH bacteria adhered together (Fig. 1E ). In addition, the overexpression of ydeH changed the colony phenotype on LB or 7H10 agar plates. The ydeH strain formed a typical wrinkled colony that was rougher than the smooth and wet colonies of the ydeH (mut) strain (Fig. 1F, G ). Fig. 1: c-di-GMP controls biofilm formation by M. smegmatis . A Adhesion of the ydeH , and ydeH (mut) strains. B Sedimentation rate of the ydeH (mut), and ydeH strains. C Pellice formation of the ydeH , and ydeH (mut) strains. D The cells morphology of the ydeH , and ydeH (mut) strains after staining with 2% crystal violet under light microscope. E Scanning electron microscopy assays of cell morphology for ydeH , and ydeH (mut) strains. The images were taken at 8000x magnification. The experiments of ( D – E ) were performed three times and the representative images were shown. F Colonial morphology of the ydeH and ydeH (mut) strains on LB agar plates. G Colonial morphology of the ydeH and ydeH (mut) strains on 7H10 agar plates. H Biofilm formation at the air–liquid surface of the wild type, ydeH and ydeH (mut) strains. I Quantitation of biofilm biomass by crystal violet staining of the wild type, ydeH and ydeH (mut) strains ( n = 3, biological replicates). Two-tailed t-tests were performed for statistical analysis (*** p = 0.0001). Data were presented as mean ± SD. The source data were provided in the Source data file. Full size image Changes in the surface morphology of bacterial colonies are often accompanied by changes in biofilm formation. We further investigated the effect of c-di-GMP on biofilm formation in M. smegmatis . As shown in Fig. 1H , the ydeH strain formed a strong biofilm and denser structured pellicle at the air–liquid surface when cultured in modified M63 medium. In contrast, the ydeH (mut) and WT strains exhibited sparse structured pellicles. The results were consistent with the biofilm biomass assay with crystal violet staining (Fig. 1I ). And there was no significant difference in the growth of WT, ydeH, and ydeH (mut) strains, indicating that the biofilm formation was not related to the growth (Fig. S1A ). Biofilm formation is associated with the motility of bacteria [21] , [29] , so the motility of the WT, ydeH and ydeH (mut) strains was further investigated on semisolid M63 medium. The motility of the ydeH strain was reduced compared to that of the WT and ydeH (mut) strains (Fig. S2 ). In conclusion, our results indicate that high levels of c-di-GMP can increase adhesion and sedimentation, alter wrinkled colonies, promote biofilm formation, and inhibit the motility of M. smegmatis . c-di-GMP affects biofilm formation in a manner dependent on Lsr2 Msm in M. smegmatis To investigate the regulatory mechanism of c-di-GMP on biofilm formation and identify the effector, we generated a transposon insertion mutant library of M. smegmatis with high levels of c-di-GMP. DNA sequencing and analysis of a colony-altered mutant revealed that a transposon was inserted into the lsr2 Msm gene (MSMEG_6092). Therefore, we speculate that c-di-GMP may regulate biofilm formation through Lsr2 Msm , a nucleoid‑associated protein (NAP). To confirm our hypothesis, we constructed an lsr2 Msm deletion mutant strain (verified by RT-qPCR, Fig. S3 ) and several recombinant strains by complementing the lsr2 Msm gene or overexpressing the ydeH gene in the lsr2 Msm KO strain ( lsr2 Msm Com and lsr2 Msm KO/ ydeH ), with the lsr2 Msm deletion mutant strain had an empty pMV261 vector as a control ( lsr2 Msm KO). As shown in Fig. S4A–C , the colony phenotype of the lsr2 Msm com strain was partially restored to that of the WT strain. There was no significant difference in biofilm formation or quantitative biofilm biomass between the lsr2 Msm com and WT strains. The rough colony ydeH- overexpressing strains formed stronger biofilms than the smooth colony lsr2 Msm KO strain, which formed a very weak biofilm (Fig. 2A–C ). The lsr2 Msm KO/ ydeH strain formed a smooth colony and poor biofilm similar to those of the lsr2 Msm KO strain (Fig. 2A–C ). This result was consistent with the quantitative biofilm biomass results of crystal violet staining (Fig. 2D ). And there was no significant difference in the growth of these strains, indicating that the biofilm formation was not related to the growth (Fig. S1B, C ). These indicate that high levels of c-di-GMP can significantly alter the colony surface morphology of the WT strain of M. smegmatis but have no effect on the lsr2 Msm KO strain. In addition, we constructed the recombinant strains with downregulated gene expression using the CRISPRi (verified by RT-qPCR, Fig. S5 ) to examine the effect of other receptors of c-di-GMP including DevR Msm and LtmA Msm on colony morphology and biofilm formation in M. smegmatis . The results show that there were no significant difference in growth, colony morphology and biofilm formation among the pLJR962, devR Msm CRISPRi and ltmA Msm CRISPRi strains (Figs. S1 D and S6 ). Fig. 2: c-di-GMP control biofilm formation via Lsr2 Msm , and Lsr2 Msm is a c-di-GMP receptor. A Spot colony morphology of the wide type, lsr2 Msm knock-out and lsr2 Msm KO/ ydeH strains. B Single colony morphology of the ydeH , lsr2 Msm KO and lsr2 Msm KO/ ydeH strains on 7H10 medium. C Biofilm formation at the air–liquid surface of the ydeH , lsr2 Msm KO and lsr2 Msm KO/ ydeH strains. D Biofilm biomass quantitation of the ydeH , lsr2 Msm KO and lsr2 Msm KO/ ydeH strains by crystal violet staining ( n = 3, biological replicates). Two-tailed t-tests were performed for statistical analysis (*** p = 0.0002). Data were presented as mean ± SD. E ITC assays for the interaction between Lsr2 Msm and c-di-GMP. Original titration data and integrated heat measurements were shown in the upper and lower plots. The source data were provided in the Source data file. Full size image Therefore, our data suggest that c-di-GMP largely relies on the NAP Lsr2 Msm to regulate colony phenotype and biofilm formation in M. smegmatis . Lsr2 Msm is a c-di-GMP receptor As a signaling molecule, c-di-GMP exerts its function through its downstream receptor, while it regulates biofilm formation in a manner dependent on Lsr2 Msm . Therefore, Lsr2 Msm might be a potential receptor for c-di-GMP, and we further validated this possibility through an isothermal titration calorimetry (ITC) assay. As shown in Fig. 2E , the raw data for titration of c-di-GMP against Lsr2 Msm indicating that the interaction is exothermic (upper plots). The integrated heat measurements were shown in the lower plots. The binding stoichiometry between c-di-GMP and Lsr2 Msm was 1:1 ( n = 0.869 ± 0.03), and the binding affinity of the interaction (Kd) was 9.644 × 10 −8 ± 0.17 M. This result demonstrates that Lsr2 Msm can directly interact with c-di-GMP and that Lsr2 Msm is a receptor for c-di-GMP to control biofilm formation. hadD Msm positively regulates biofilm formation in M. smegmatis To further explore the regulatory pathway by which c-di-GMP and Lsr2 Msm control biofilm formation, we constructed a whole-genome CRISPRi library using the dCas9- sgRNA complex to target and repress gene expression in high c-di-GMP-content M. smegmatis [30] , [31] . A recombinant strain ( hadD Msm CRISPRi) with a significantly altered colony morphology was screened on 200 ng/mL anhydrotetracycline (ATc) plates (Fig. S7 ), and further sequencing revealed that the gene target with CRISPRi was hadD Msm (MSMEG_0948). HadD Msm is a 3R-hydroxyacyl-ACP dehydratase of the type II fatty acid synthase group that catalyzes the elongation step during MA biosynthesis [26] . The colony phenotype of the hadD Msm deletion strain ( hadD Msm KO) and complementary strain ( hadD Msm Com) further confirmed that the altered colony phenotype was caused by the deletion of hadD Msm (Fig. S8A ). Furthermore, as shown in Fig. 3A , the hadD Msm KO strain exhibited a smooth colony similar to that of the lsr2 Msm KO strain, and the hadD Msm complementary strain morphology was restored to the WT phenotype. In addition, biofilm formation observation and quantitation for these three strains showed that the hadD Msm deletion mutant formed a fragile biofilm after a delay, and the WT and hadD Msm Com strains exhibited significant wrinkled pellicle biofilm formation (Fig. S8B, C ). And there was no significant difference in the growth of these strains, indicating that the biofilm formation was not related to the growth (Fig. S1E ). Fig. 3: Lsr2 Msm regulates biofilm formation in a manner dependent on hadD Msm . A Spot colony morphology of the WT, hadD Msm KO and its hadD Msm complementary strains. B EMSA assays for the hadD Msm promoter DNA-binding activity of Lsr2 Msm . hadD Msm p was co-incubated with increasing amounts of Lsr2 Msm (lanes 2–5). The experiment was performed three times and the representative image was shown. C The β-galactosidase activity experiment to assay for the effect of the Lsr2 Msm on the expression of hadD by overexpressing hadD Msm p- lacZ plasmid in the wild-type M. smegmatis strain (Msm/WT) and lsr2 Msm knock-out strain ( lsr2 Msm KO) ( n = 3, biological replicates). None promoter- lacZ and hsp60 p- lacZ were used as controls. The data were presented as Miller units on the right panel. Left column: schematic representation of each plasmid used to construct recombinant strains. Two-tailed Student’s t-tests were performed for statistical analysis of three independent biological experiments (* p = 0.0011). D Biofilm formation at the air–liquid surface of the WT, lsr2 Msm KO, hadD Msm KO and its lsr2 Msm overexpression strains. E Quantitation of biofilm biomass by crystal violet staining ( n = 3, biological replicates). Two-tailed t-tests were performed for statistical analysis (** p = 0.0023). F The quantity of keto-MA between the WT and lsr2 Msm KO M. smegmatis strains detected by lipidomic assays ( n = 6, biological replicates). The significant differences were determined by unpaired two-tailed Student’s t-test (** p = 0.0024, ** p = 0.0033). Data were presented as mean ± SD of ( C ), ( D ), ( F ). The source data were provided in the Source data file. Full size image These results indicate that hadD Msm is important for biofilm formation in M. smegmatis . Lsr2 Msm positively regulates biofilm formation by directly regulating hadD Msm Lsr2 Msm and hadD Msm perform similar functions in regulating biofilm formation and Lsr2 Msm is a NAP with extensive regulatory functions. Therefore, we hypothesized that Lsr2 Msm affects biofilm formation through its regulatory effect on hadD Msm . To verify our hypothesis, an EMSA conducted in vitro confirmed that Lsr2 Msm could directly regulate hadD Msm (Figs. 3B and S9 ). In contrast, Lsr2 Msm mutant protein loses the DNA-binding activity (Fig. S10A, B ). A β-galactosidase activity assay was conducted to further characterize the regulatory effect of Lsr2 Msm on the expression of hadD Msm . The expression level of hadD Msm p- lacZ in the WT strain was significantly higher than that in the lsr2 Msm KO strain (Fig. 3C ). However, there was no significant difference between the WT and lsr2 Msm KO strains in the expression of lacZ when the irrelevant control, ms5038 p and ms4718 p, were used as promoters (Fig. S11 ). These results indicate that Lsr2 Msm directly positively regulates the transcription of hadD Msm . Next, we further identified whether Lsr2 Msm controls biofilm formation by regulating hadD Msm . lsr2 Msm was overexpressed in the hadD Msm deletion mutant ( hadD Msm KO/ lsr2 Msm OE) for colony morphology and biofilm detection. Notably, the hadD Msm KO/ lsr2 Msm OE strain exhibited a smooth colony phenotype similar to that of the hadD Msm KO and lsr2 Msm KO strains (Fig. S12A, B ). Furthermore, the three strains formed fragile biofilms at the air–liquid interface, and their biofilm biomass was significantly lower than that of the WT strain (Fig. 3D, E ). And there was no significant difference in the growth of these strains, indicating that the biofilm formation was not related to the growth (Fig. S1F ). Lsr2 Msm positively regulated biofilm formation, but the overexpression of lsr2 Msm had no effect on biofilm formation of the hadD Msm KO/ lsr2 Msm OE strain due to the deletion of hadD Msm . In conclusion, these results indicate that Lsr2 Msm regulates biofilm formation by directly upregulating the expression of hadD Msm . Lsr2 Msm regulates keto-MA synthesis to control biofilm formation in M. smegmatis Lsr2 Msm is involved in biofilm formation. To analyze the role of Lsr2 Msm in biofilm formation in depth, lipidomic analysis was performed on the lsr2 Msm KO strain. As shown in Fig. S13 , significant changes were detected in the levels of 484 molecules, among which 241 molecules were significantly enriched in the lsr2 Msm KO strain (fold change >1.2, p < 0.05), and 243 molecules were significantly depleted (fold change <0.83, p < 0.05) compared with the WT strain. Further analysis showed that in the lsr2 Msm deletion mutant, keto-MA (C78, C80) were significantly depleted (Fig. 3F ). This result was consistent with the decrease in the context of long-chain keto-MA in the hadD- deficient strain, which resulted in poor biofilm formation, as previously reported [27] . In general, our data suggest that Lsr2 Msm regulates the synthesis of keto-MA by hadD Msm to control biofilm formation. c-di-GMP relies on hadD Msm to regulate biofilm formation in M. smegmatis hadD Msm is a target gene directly regulated by Lsr2 Msm , and Lsr2 Msm is a c-di-GMP receptor that regulates biofilm formation. Next, we investigated whether the regulation of biofilm formation by c-di-GMP depends on the hadD Msm gene. An ydeH overexpression strain was constructed bearing the hadD Msm deletion mutation ( hadD Msm KO/ ydeH ). The colony phenotype results showed that hadD Msm KO/ ydeH strain formed a smoother colony than the WT strain and a rougher colony than the hadD Msm KO strain. In contrast, the ydeH strain formed the roughest colony (Figs. 4 A and S14 ). Biofilm formation and quantitation assays showed that the ydeH strain formed robust biofilms, but the hadD Msm KO and hadD Msm KO/ ydeH strains formed weak biofilms (Fig. 4B, C ). And there was no significant difference in the growth of these strains, indicating that the biofilm formation was not related to the growth (Fig. S1G ). The expression of ydeH did not restore biofilm formation in the hadD Msm KO strain, indicating the key role of hadD Msm in this pathway. Fig. 4: c-di-GMP promotes the expression of hadD Msm by Lsr2 Msm to affect biofilm formation in M. smegmatis . A Spot colony morphology of the wide type and its ydeH -overexpressed strains, hadD Msm knock-out and its ydeH -overexpression strains. B Biofilm formation of the WT, ydeH , hadD Msm KO, and hadD Msm KO/ ydeH strains. C Quantitation of biofilm biomass by crystal violet staining of the WT, ydeH , hadD Msm KO, and hadD Msm KO/ ydeH strains ( n = 3, biological replicates). Two-tailed t-tests were performed for statistical analysis (*** p = 0.0004). D RT-PCR quantitation of hadD Msm transcription in the ydeH , ydeH (mut)-overexpressed M. smegmatis strains. Two-tailed Student’s t-tests were performed for statistical analysis (**** p < 0.0001). RT-PCR and gel analysis were performed under the same conditions and each experiment was performed three independent biological replicates. no RT was genomic DNA contamination control. E ChIP assays for the effect of c-di-GMP on the intracellular hadD Msm p-binding activity of Lsr2 Msm in M. smegmatis . The input (5%) indicated that the supernatant of disrupted cells was diluted to 5%, ChIP using preimmune (P) or immune (I) sera raised against HisLsr2 Msm . DNA of the input (5%), P, and I were used as temples for PCR (the right panel) ( n = 3, biological replicates) and RT-qPCR (the light panel). M: DNA Marker. Two-tailed Student’s t-tests were performed for statistical analysis (**** p < 0.0001). F β-galactosidase activity assays. The effect of c-di-GMP on Lsr2 Msm regulates the expression of hadD Msm was assayed by overexpressing pMV261- hadD Msm p- ydeH - lacZ and pMV261- hadD Msm p- ydeH (mut)- lacZ plasmids in the Msm/WT, lsr2 Msm KO strains ( n = 3, biological replicates). None promoter- lacZ and hsp60 p- lacZ plasmids overexpression were used as controls. Two-tailed Student’s t-tests were performed for statistical analysis (* p = 0.0414, **** p < 0.0001). Data were presented as mean ± SD of ( C ), ( D ), ( E ), ( F ). The source data were provided in the Source data file. Full size image Here, we characterized that the contribution of hadD Msm to the c-di-GMP-dependent regulation of colony morphology and biofilm formation of M. smegmatis and showed that hadD Msm is a necessary gene for c-di-GMP-mediated to regulation of the biofilm formation pathway. c-di-GMP activates Lsr2 Msm to upregulate the expression of hadD Msm in M. smegmatis Our previous results showed that hadD Msm was the essential gene for c-di-GMP and Lsr2 Msm to regulate biofilm formation. Therefore, we hypothesized that c-di-GMP controls biofilm formation by regulating the transcription of hadD Msm via Lsr2 Msm . The impact of c-di-GMP on the expression level of hadD Msm was examined through RT‒PCR. As shown in Fig. 4D , hadD Msm was significantly upregulated in the ydeH strain compared to the ydeH (mut) strain (Fig. 4D ), indicating that high levels of c-di-GMP activated the expression of hadD Msm . This might be due to the influence of c-di-GMP on the regulation of hadD Msm by Lsr2 Msm . Furthermore, we demonstrated that increasing amounts of c-di-GMP (0.8–16 μM) stimulates the DNA-binding activity of Lsr2 Msm through EMSA assays (Fig. S15 ). To further clarify the regulatory relationship, a chromatin immunoprecipitation (ChIP) assay was conducted to verify whether high levels of c-di-GMP affect the hadD Msm p-binding activity of Lsr2 Msm . His-Lsr2 Msm and the ydeH gene were co-overexpressed in WT M. smegmatis to construct a high c-di-GMP-content strain (Msm/ hislsr2 Msm - ydeH ), and ydeH (mut) was co-overexpressed to construct a control strain (Msm/ hislsr2 Msm - ydeH (mut)). As shown in Fig. 4E , the amount of hadD Msm p precipitated by Lsr2 Msm from the hislsr2 Msm - ydeH- overexpressing strain was significantly higher than that precipitated from the hislsr2 Msm - ydeH (mut)-overexpressing strain. Our results indicated that high levels of c-di-GMP significantly activated the hadD Msm p-binding activity of Lsr2 Msm in M. smegmatis . The effect of intracellular c-di-GMP on the Lsr2 Msm regulation of hadD Msm was further verified by a β-galactosidase activity assay. We constructed hadD Msm p- ydeH (mut)- lacZ or hadD Msm p- ydeH - lacZ coexpression plasmids and inserted them into WT and lsr2 Msm KO strains by transformation. Interestingly, the expression of lacZ by the hadD Msm p- ydeH overexpression construct in the WT strain was higher than that of the overexpression construct in the lsr2 Msm KO strain. The expression of lacZ in the hadD Msm p- ydeH -overexpressing WT strain was significantly upregulated compared with that in the hadD Msm p- ydeH (mut)-overexpressing WT strain (Fig. 4F ). These results indicated that c-di-GMP enhanced the expression of hadD Msm through Lsr2 Msm . In summary, our data suggest that c-di-GMP promotes biofilm formation by activating the hadD Msm p-binding activity of Lsr2 Msm to upregulate the expression of hadD Msm in M. smegmatis . Lsr2 is a conserved c-di-GMP receptor, and the regulation of biofilm formation by lsr2 and hadD is conserved in mycobacteria Lsr2 is a well-known NAP in M. tuberculosis and M. smegmatis [16] , [24] , [32] . Sequence analysis revealed that Lsr2 is conserved in several important mycobacterial species ( M. tuberculosis , M. bovis BCG, and M. smegmatis ) (Fig. S16A ). The ITC assay showed the specific binding curve of Lsr2 Mtb and c-di-GMP, indicating that Lsr2 Mtb was also a c-di-GMP signaling receptor in M. tuberculosis . The binding stoichiometry between Lsr2 Mtb and c-di-GMP was 1:1 (0.923 ± 0.07), and the binding affinity of the interaction (Kd) was 1.074 × 10 −7 ± 0.14 M (Fig. 5A ). Fig. 5: The c-di-GMP signal regulatory system is conserved in mycobacteria including M. tuberculosis . A ITC assays for the interaction between Lsr2 Mtb and c-di-GMP. Original titration data and integrated heat measurements are shown in the upper and lower plots. B Spot colony morphology of the wide type, hadD Msm knock-out and hadD Mtb complementary strains. C Biofilm formation of the WT, hadD Msm KO, and hadD Mtb complementary strains. D Quantitation of biofilm biomass of the WT, hadD Msm KO, and hadD Mtb complementary strains by crystal violet staining ( n = 3, biological replicates). Two-tailed t-tests were performed for statistical analysis (**** p < 0.0001, *** p = 0.0004). E EMSA assays for the effect of c-di-GMP on hadD BCG promoter DNA-binding activity of Lsr2 BCG . hadD BCG p was co-incubated with increasing concentration of Lsr2 BCG (lanes 2–5). Three independent experiments were performed. F RT-PCR for transcriptional analysis of hadD BCG in the WT, lsr2 BCG KO M. bovis BCG strains ( n = 3, biological replicates). Two-tailed Student’s t-tests were performed for statistical analysis (**** p < 0.0001). RT-PCR and gel analysis were performed under the same conditions. G Spot colony morphology of the WT and lsr2 BCG knock-out BCG strains on 7H10 plates. H RT-PCR for transcriptional analysis of hadD BCG in the ydeH (mut), ydeH -overexpressed M. bovis BCG strains ( n = 3, biological replicates). Two-tailed Student’s t-tests were performed for statistical analysis (**** p < 0.0001). I ChIP assays for the effect of c-di-GMP on the intracellular DNA-binding activity of Lsr2 BCG in the M. bovis BCG strains. The input (5%) indicated that the supernatant of disrupted cells was diluted to 5%, ChIP using preimmune (P) or immune (I) sera raised against HisLsr2 BCG . DNA sample of the input (5%), P, and I were used as temples for PCR (the right panel) ( n = 3, biological replicates) and were quantified using RT-qPCR (the light panel). M: DNA marker. Two-tailed Student’s t-tests were performed to for statistical analysis (**** p < 0.0001). Data of figures ( D ), ( F ), ( H ), and ( I ) were presented as mean ± SD. The source data were provided in the Source data file. Full size image Next, we further showed that hadD is highly conserved among important mycobacterial species (Fig. S16B ). The HadD protein is encoded by rv0504 , and bcg0547 is entirely identical in M. tuberculosis and M. bovis BCG, sharing 65.2% identity with hadD Msm . Previous reports and our results confirmed that the regulation of colony morphology and biofilm formation by hadD Msm is conserved [26] , [27] . The smooth colony phenotype of the hadD Msm KO strain was partially restored to the WT phenotype with the introduction of hadD Mtb of M. tuberculosis ( hadD Msm KO/ hadD Mtb Com) (Figs. 5B , S16C ). The results of biofilm culture and quantification are consistent with these findings (Fig. 5C, D ). And there was no significant difference in the growth of these strains, indicating that the biofilm formation was not related to the growth (Fig. S1H ). In conclusion, as a receptor for c-di-GMP, NAP Lsr2 is conserved in mycobacteria. In addition, hadD from M. tuberculosis and M. smegmatis relatively conservatively regulates biofilm formation. Lsr2 regulates biofilm formation by positively regulating the expression of hadD in M. bovis BCG Next, we used the vaccine strain M. bovis BCG to investigate the effect of Lsr2 BCG regulation of hadD BCG on biofilm formation. First, an EMSA demonstrated that Lsr2 BCG bound well to hadD BCG p (Figs. 5E and S17 ). In contrast, Lsr2 Mtb mutant protein loses the DNA-binding activity (Fig. S18 ). Then, RT‒PCR results showed that the expression of hadD BCG was obviously reduced in the lsr2 BCG -deficient mutant ( lsr2 BCG KO) strain (verified by RT‒qPCR, Fig. S19 ) compared to that in the WT M. bovis BCG strain (Fig. 5F ). Finally, the smooth colony phenotype of the lsr2 BCG KO strain indicated that Lsr2 BCG regulated the colony phenotype in M. bovis BCG (Fig. 5G ). These data indicate that Lsr2 directly stimulates the expression of hadD to control colony morphology and biofilm formation in a conserved manner. c-di-GMP promotes positive regulation of hadD BCG expression by Lsr2 Upon finding the conserved regulation of hadD BCG by Lsr2 BCG to control biofilm formation, we further investigated whether the effect of c-di-GMP on this regulation is conserved in the M. bovis BCG strain. We significantly increased the intracellular levels of c-di-GMP in M. bovis BCG through overexpressing ydeH from E. coli (Fig. S20 ) [28] . RT‒PCR results showed that the expression level of hadD BCG significantly increased in the ydeH -overexpressing M. bovis BCG strain (BCG/ ydeH ) (Fig. 5H ). This result indicates that a high level of c-di-GMP triggers the expression of hadD BCG in M. bovis BCG. ChIP assays were conducted to confirm the regulatory effect of high levels of c-di-GMP on the DNA-binding activity of Lsr2 BCG in M. bovis BCG . We overexpressed hislsr2 BCG and ydeH via the pMV261 plasmid to produce a high level of c-di-GMP in the WT M. bovis BCG strain (BCG/ hislsr2 BCG - ydeH ) and overexpressed hislsr2 BCG and ydeH (mut) to construct a control strain (BCG/ hislsr2 BCG - ydeH (mut)). As shown in Fig. 5I , Lsr2 BCG precipitated ~3 times the hadD BCG promoter from the hislsr2 BCG - ydeH -overexpressing strain compared to that from the hislsr2 BCG - ydeH (mut)-overexpressing strain. Therefore, this result indicated that high levels of c-di-GMP could significantly promote the hadD BCG p-binding activity of Lsr2 BCG in M. bovis BCG . Taken together, these findings suggest that a high level of c-di-GMP activates Lsr2 to positively regulate the expression of hadD in mycobacteria. Moreover, the increased synthesis of keto-MA contributing to biofilm formation is conserved in mycobacteria, including the important M. tuberculosis and M. bovis BCG strains. Bacteria preferentially transform from suspension culture to a biofilm mode of growth under high levels of c-di-GMP [33] . However, the regulatory pathway of c-di-GMP regulation of biofilm formation in mycobacteria has not been reported. In this study, we report that the robust biofilm formation induced by c-di-GMP depends on the receptor Lsr2, which is a NAP. We successfully demonstrated that Lsr2 positively regulates hadD to regulate biofilm formation. Our data revealed that c-di-GMP could bind to Lsr2 at a ratio of 1:1 and enhance the positive regulation of hadD expression by Lsr2. HadD is involved in the synthesis of keto-MA and contributes to biofilm formation. We revealed the complete regulatory pathway by which c-di-GMP regulated robust biofilm formation through Lsr2 to affect lipid synthesis. This is also the report of a NAP that plays a role in c-di-GMP functional regulation in mycobacteria. Since the discovery of the c-di-GMP receptor, multiple regulatory mechanisms of c-di-GMP in diverse bacterial processes have been extensively reported [2] , [5] , [34] . In recent years, several c-di-GMP receptors and their physiological regulatory functions in mycobacteria have been confirmed [35] . The c-di-GMP effector, LtmA, stimulates the expression of 37 lipid transport and metabolism genes in M. smegmatis [28] . Another c-di-GMP receptor, HpoR, acts as an inhibitor to enhance mycobacterial antioxidant defense [36] . Interestingly, c-di-GMP can integrate LtmA and HpoR to regulate antioxidant processes [36] . In addition, the two-component regulator DevR was characterized as a new c-di-GMP receptor in response to oxidative stress [37] . Here, we found that NAP Lsr2 is a receptor of c-di-GMP that regulates mycobacterial biofilm formation. Lsr2 is a known global transcriptional regulator that contributes to multiple physiological processes [17] , [18] , [19] , [23] , [24] . Therefore, our findings indicated that c-di-GMP could combine with NAP Lsr2 to perform wide regulatory functions in mycobacteria. Biofilms are well known to contribute to the drug resistance of bacteria [38] , chronic infections [39] , [40] , and persistent infections [41] , [42] by pathogenic bacteria. For example, Pseudomonas aeruginosa mucoid strains form biofilms in the lungs, leading to cystic fibrosis [43] . 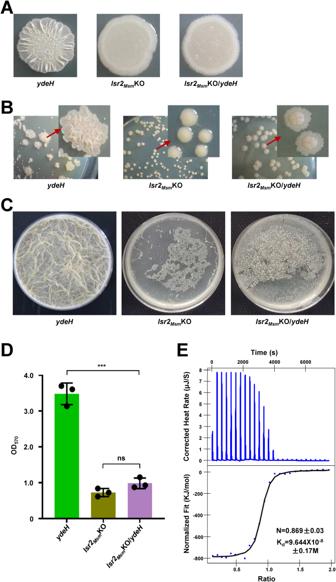Fig. 2: c-di-GMP control biofilm formation via Lsr2Msm, and Lsr2Msmis a c-di-GMP receptor. ASpot colony morphology of the wide type,lsr2Msmknock-out andlsr2MsmKO/ydeHstrains.BSingle colony morphology of theydeH,lsr2MsmKO andlsr2MsmKO/ydeHstrains on 7H10 medium.CBiofilm formation at the air–liquid surface of theydeH,lsr2MsmKO andlsr2MsmKO/ydeHstrains.DBiofilm biomass quantitation of theydeH,lsr2MsmKO andlsr2MsmKO/ydeHstrains by crystal violet staining (n= 3, biological replicates). Two-tailed t-tests were performed for statistical analysis (***p= 0.0002). Data were presented as mean ± SD.EITC assays for the interaction between Lsr2Msmand c-di-GMP. Original titration data and integrated heat measurements were shown in the upper and lower plots. The source data were provided in the Source data file. M. tuberculosis is the causal agent of TB. Chronic TB is difficult to treat with current first-line anti-TB drugs owing to the emergence of multidrug-resistant bacteria. Part of the reason is the formation of biofilms by M. tuberculosis in the lung [44] , [45] . Therefore, target genes involved in biofilm formation are expected to be the focus of TB treatment. In the present study, we identified the regulatory mechanism by which Lsr2 regulates mycobacterial biofilm formation. Lsr2 increases the synthesis of keto-MA in association with biofilm formation by positively regulating the expression of the target gene hadD . Importantly, high levels of c-di-GMP trigger the positive regulation of the expression of hadD by Lsr2, and the increase in keto-MA synthesis further contributes to robust biofilm formation. Thus, our research indicates that the target gene hadD is a key target for drug design for TB prevention and treatment. Overall, our current data showed that the NAP Lsr2 is a conserved c-di-GMP receptor that regulates biofilm formation in mycobacteria. c-di-GMP positively regulates the expression of hadD via Lsr2 to affect biofilm formation, and this pathway is conserved in mycobacteria. Our findings support the model shown in Fig. 6 . The increase in the c-di-GMP signal level promotes the positive regulation of hadD by Lsr2, leading to an increase in the synthesis of keto-MA. Thereafter, keto-MA can be converted into trehalose monomycolate (TMM) and trehalose dimycolate (TDM) [46] . TMM, TDM, and MA are important components of the cell wall and affect mycobacterial biofilm formation [26] , [47] . Our findings extend the regulatory function of c-di-GMP to biofilm formation in mycobacteria. This research also provides a reference for further studies of the extensive signaling pathways of c-di-GMP through NAP. Fig. 6 The model of which c-di-GMP stimulates the expression of hadD by Lsr2 to control biofilm formation in mycobacteria. Full size image Expression and purification of recombinant proteins lsr2 genes were amplified from genomic DNA of the M. smegmatis mc 2 155 and M. tuberculosis strains by polymerase chain reaction (PCR) using appropriate primer pairs (Tsingke Biotech, Beijing). The amplified DNA fragments were cloned into modified pET28a expression vector to obtain recombinant plasmids that were introduced into E. coli BL21 (DE3) cells. The cells were cultured to an optical density at 600 nm (OD 600 ) of 0.6 in 200 mL LB medium (Trytone 20 g/L (#LP0042B, OXOID), Yeast Extract 10 g/L (#LP0021B, OXOID), NaCl 20 g/L (#A501218, Sangon Biotech)). Protein expression was induced by addition of 0.4 mM isopropyl-β-D-1-thiogalactopyranoside (IPTG) (#I8070, Solarbio) for 12 h at 16 °C. The cells were collected by centrifugation and the protein (His-tag at the C-terminal) was purified by affinity chromatography on Ni-NTA agarose (#SA05101L, Smart-Lifesciences) [28] , [36] . The column-bound protein was washed with a wash buffer (100 mM Tris–HCl (#T1503, Sigma) pH 8.0, 500 mM NaCl and 40 mM imidazole (#I8090, Solarbio)) and dialyzed using an elution buffer (100 mM Tris–HCl pH 8.0, 500 mM NaCl and 250 mM imidazole). The protein was stored at −80 °C. Purified proteins were verified by sodium dodecyl sulfate-polyacrylamide gel Electrophoresis (SDS-PAGE). Protein concentration was detected by the Bradford method and Nano Drop (Thermo Fisher, USA). Generation of a high-level c-di-GMP transposon M. smegmatis library and screening the target genes of c-di-GMP The DGC gene ydeH from Escherichia coli was cloned and inserted into a modified pMV261 plasmid containing a hygromycin resistance gene to obtain a recombinant plasmid. Subsequently, the recombinant plasmid was introduced into M. smegmatis mc 2 155 by transformation to obtain a high c-di-GMP-content M. smegmatis strain ( ydeH ). Then, the transposon system containing a kanamycin resistance gene was introduced into the ydeH strain to generate a transposon insertion mutant library of high levels of c-di-GMP of M. smegmatis as described previously. The cells of the transposon insertion mutant library were coated on 7H10 agar medium (#262710, BD Difco) supplemented with 0.5% (v/v) glycerol (#A600232, Sangon Biotech), kanamycin (Kan) (#I8020, Solarbio) and hygromycin (Hyg) (#H8080, Solarbio) and cultured at 37 °C for 3–5 days. The strains with altered colony morphology were isolated and cultured in 7H9 medium (#271310, BD Difco) supplemented with 0.2% (v/v) glycerol and 0.05% (v/v) Tween-80 (#A600562, Sangon Biotech) to OD 600 1.2. The cells were collected, and genomic DNA was extracted with a bacterial genome extraction kit (#DN1101, Aidlab). Furthermore, the sequences near the insertion site of the transposon were amplified by thermal asymmetric PCR and sequenced to analyze the location of the transposon [19] , [48] . The primers for ydeH overexpression and transposon insertion mutant sequence analysis are shown in the Source data file (Primer list). Construction of the deletion mutants and complementation mycobacteria lsr2 and hadD genes were knocked out by a gene replacement strategy [49] . Upstream and downstream fragments of lsr2 Msm , hadD Msm , and lsr2 BCG were amplified using corresponding primer pairs. The amplified DNA fragments were cloned into a pMind-derived suicide plasmid that carried a hygromycin resistance gene and a lacZ selection market. Subsequently, these recombinant plasmids were inserted into mycobacteria by transformation. lsr2 Msm , hadD Msm , and lsr2 BCG knock-out strains were selected and identified with PCR [50] . The complementation strains were generated using plasmid pMV261. The primers for genes knockout and complementation were shown in the Source data file (Primer list). Morphological observation Mycobacteria for morphological observation was grown to a mid-log phase (OD 600 1.0–1.2) in 7H9 medium. The cells were collected by centrifuge and washed with PBS. Next, the cells were re-suspended in 1 mL 25% glutaraldehyde (#G5882, Sigma-Aldrich) and fixed overnight at 4 °C. Then, the cells were freeze-dried after beening dehydrated by ethanol (#A500737, Sangon Biotech). The cells were fixed on the conductive tape and observed by Quattro scanning electron microscopy (OPTON, China) [51] . The cells of crystal violet staining were observed using OLYMPUS CX33 optical microscope (Olympus Corporation, Japan). Mycobacterial colony morphologies were investigated by spot-inoculating 2 μL cultures in 7H10 or LB agar medium at 37 °C for 3–5 days to observe colony morphology. Cultures were diluted to a concentration of 10 6 in 100 μL and were plated on 7H10 agar medium to observe single colony morphology. Biofilm formation and quantitative analysis Biofilm formation was performed referring to the previously described procedures [13] . Mycobacteria was cultured to OD 600 1.0–1.2 in 7H9 medium and was suspended in a modified M63 medium (addition of 1% (w/v) glucose (#G8150, Solarbio), 0.5% (w/v) casamino acid (#C822594, Macklin), 1 mM MgSO 4 (#20025118, Sinopharm) and 0.7 mM CaCl 2 ) (#10005861, Sinopharm)). 5 mL of mycobacterial suspension with an OD 600 of 0.3 was inoculated into a 12-well PVC microtiter dishes and was incubated at 30 °C without shaking for 5 days to observe biofilms formation at gas–liquid surface. 100 μL mycobacterial suspension with an OD 600 of 0.1 was used to quantify the biofilm formation by crystal violet staining assay [10] , [48] . Mycobacterial suspension was incubated for 48 h at 37 °C with shaking at 80 rpm in 96-well PVC microtiter dishes. Biofilms were stained with 1% (w/v) crystal violet (CV) (#C8470, Solarbio) at room temperature for 30 min and were extracted with ethanol (#A500737, Sangon Biotech)/acetone (#W332615, Sigma-Aldrich) (v/v = 80:20). The extracted biofilms were measured at OD 570 using a TECAN Infinite M200 Pro Nano Quant microplate reader (Mannedorf, Switzerland). Screening downstream target genes of c-di-GMP by the CRISPRi platform CRISPRi platform was constructed through using the plasmid pLJR962 [31] . sgRNA scaffolds targeting the M. smegmatis genome were designed with two unique Bsm B I (#R0739L, NEB) restriction sites. Then, the complementary sgRNA oligos were annealed and ligated into the CRISPRi vector backbone (pLJR962) to construct CRISPRi plasmids. The mixed CRISPRi plasmids of the M. smegmatis genome were inserted into the high c-di-GMP-content M. smegmatis strain via transformed, and the resulted strains were cultured on 7H10 plates containing 200 ng/mL ATc (#IA5330, Solarbio) for 3–5 days at 37 °C. The empty pLJR962 vector was inserted into the high c-di-GMP-content M. smegmatis strain via transformation as a control (pLJR962). The change in the colony phenotype of M. smegmatis strain was screened and sequenced with a primer pair to confirm the gene targeting by dCas9-sgRNA complex. RNA extraction and RT-PCR assay Mycobacteria cells were grown to OD 600 1.0–1.2 in 7H9 medium and their RNA were extracted by using the RNA extraction kit (#RN0802, Aidlab). 500 ng total RNA was reverse transcribed to cDNA by using a TRUEscript strand cDNA synthesis kit (#PC1803, Aidlab). cDNA was used as a template for RT-PCR to analysis the expression of target gene. RT-PCR assay was performed using a 25 μL conventional PCR reaction and the following protocol: predenaturation at 95 °C for 5 min, 40 cycles of 95 °C for 10 s, 60 °C for 30 s, 72 °C for 30 s, and annealing at 72 °C for 5 min. PCR products were analysis by loading on 1.5% agarose (#BY-R0100, Biowest) gel electrophoresis. Images were acquired by a Geldoc scanner (Bio-Rad, USA). The source data were provided in the Source Data file. The primers used in RT-PCR assay were listed in the Source Data file (Primer list). Electrophoretic mobility shift assay (EMSA) The upstream regulatory sequence of lsr2 or hadD clusters used in electrophoretic mobility shift assay (EMSA) were amplified from mycobacterial genome by PCR. Primer pairs for PCR were listed in the Source data file (Primer list). EMSA assays were conducted to detect the hadD promoter-binding activity of Lsr2 [50] , [52] DNA fragments were co-incubated with various concentration of protein diluted in a buffer (50 mM Tris–HCl, pH 7.5, 10% glycerol, 50 mM NaCl) to a total volume of 30 μL at room temperature for 15 min. The mixture was directly loaded on 8% native polyacrylamide gel (#A1020, Solarbio) and separated in a buffer containing 0.5 × Tris-borate-ethylenediaminetetraacetic acid (EDTA) (#E8030, Solarbio) at 150 V for 1 h. Images were acquired by Geldoc scanner (Bio-Rad, USA). c-di-GMP were co-incubated with Lsr2 for 15 min before beening co-incubated with DNA fragments to investigate the effect of c-di-GMP on the interaction between Lsr2 and hadD promoter. The source data were provided in the Source data file. Chromatin immunoprecipitation assay and real-time qPCR analysis Chromatin immunoprecipitation (ChIP) assay was performed to investigate the effect of c-di-GMP on the interactions between Lsr2 and hadD promoters in vivo [53] . Mycobacteria were grown to OD 600 1.0 in 100 mL 7H9 medium, fixed with 1% formaldehyde (#A501912, Sangon Biotech) for 20 min and stopped with 0.125 M glycine (#62011516, Sinopharm) for 5 min. Crosslinked cells were harvested and washed with PBS for three times. The cells were re-suspended in 1 mL Tris-Buffer with Tween-20 and Triton X-100 (20 mM Tris–HCl, 150 mM NaCl, 0.1% Tween 20 (#A600560, BBI), 0.1% Triton X-100 (#A110694, Dimond), pH 7.5). The sample was sonicated on ice and centrifuged. 100 µL of supernatant was saved as input sample. The 900 µL supernatant was incubated with 1:2,000 dilution of mouse 6*His antibodies (#CSB-MA000011M0m, CUSABIO) or preimmune mouse serum (#NS03L, Sigma-Aldrich) for 3 h at 4 °C. Then, the complexes were immunoprecipitated with 20 µL 50% protein A agarose (#17127901, GE) for 1 h. The DNA was dissociated and recovered from the immunocomplex as the sample of ChIP and P [36] , [54] . The samples of Input, I and P were purified and analyzed by RT-PCR and real-time qPCR using SYBR qPCR Green Master Mix (#PC3301, Aidlab) on QuantStudio 3 Real-Time PCR System (Thermo Fisher, USA). The relative quantity of hadD p in ChIP was normalized to the levels of hadD p in input. The degrees of change in the levels of hadD p were calculated using the 2 −ΔΔCt method, and two-tailed Student’s t-tests were performed for statistical analysis. The primer pairs used in ChIP assay are listed in the Source data file (Primer list). β-galactosidase activity assays The β-galactosidase activity experiment was performed in the M. smegmatis strain by constructing no-promoter/promoter- lacZ , and promoter- yedH / yedH (mut)- lacZ expression plasmids based on pMV261 [55] . These plasmids were electroporated into the lsr2 Msm knock-out strain and WT M. smegmatis strain to obtain recombinant reporter strains. Recombinant strains were grown to OD 600 1.0–1.2 in 7H9 medium. The cells were collected and suspended in 600 μL Z buffer (60 mM Na 2 HPO 4 ⋅ 12H 2 O (#A501725, Sangon Biotech), 40 mM NaH 2 PO 4 ⋅ 2H 2 O (#A502805, Sangon Biotech), 10 mM KCl, 1 mM MgSO 4 (#A50119, Sangon Biotech), 50 mM β-Mercaptoethanol (#M8210, Solarbio)). 300 μL cell suspension was used to detect OD 600 . Another 300 μL cell suspension was treated with 100 μL chloroform (#13200, Thermo Fisher) and 100 μL 0.1% SDS (#S8010, Solarbio). Then, 200 μL 4 mg/mL substrate 2-nitrophenyl β-D-galactopyranoside (#O8040, Solarbio) was added for β-galactosidase activity detection, and 500 μL NaCO 3 (#A500840, Sangon Biotech) was used for stopping experiment. After centrifuging, the absorbance of 200 μL supernatant of reaction was detected at 600 nm, 420 nm, and 550 nm through a TECAN Infinite M200 Pro Nano Quant microplate reader (Mannedorf, Switzerland) [54] . The primers used in β-galactosidase activity experiment are listed in Source data file (Primer list) . Two-tailed Student’s t-tests were performed for statistical analysis. Comparative lipidomic analysis M. smegmatis strains were grown to OD 600 1.2 in 7H9 medium and harvested for bacterial lipidomic analysis. 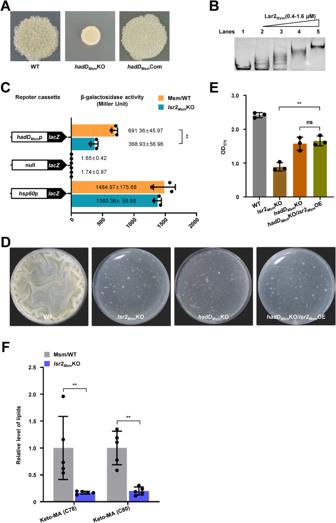Fig. 3: Lsr2Msmregulates biofilm formation in a manner dependent onhadDMsm. ASpot colony morphology of the WT,hadDMsmKO and itshadDMsmcomplementary strains.BEMSA assays for thehadDMsmpromoter DNA-binding activity of Lsr2Msm.hadDMsmp was co-incubated with increasing amounts of Lsr2Msm(lanes 2–5). The experiment was performed three times and the representative image was shown.CThe β-galactosidase activity experiment to assay for the effect of the Lsr2Msmon the expression ofhadDby overexpressinghadDMsmp-lacZplasmid in the wild-typeM. smegmatisstrain (Msm/WT) andlsr2Msmknock-out strain (lsr2MsmKO) (n= 3, biological replicates). None promoter-lacZandhsp60p-lacZwere used as controls. The data were presented as Miller units on the right panel. Left column: schematic representation of each plasmid used to construct recombinant strains. Two-tailed Student’s t-tests were performed for statistical analysis of three independent biological experiments (*p= 0.0011).DBiofilm formation at the air–liquid surface of the WT,lsr2MsmKO,hadDMsmKO and itslsr2Msmoverexpression strains.EQuantitation of biofilm biomass by crystal violet staining (n= 3, biological replicates). Two-tailed t-tests were performed for statistical analysis (**p= 0.0023).FThe quantity of keto-MA between the WT andlsr2MsmKOM. smegmatisstrains detected by lipidomic assays (n= 6, biological replicates). The significant differences were determined by unpaired two-tailed Student’s t-test (**p= 0.0024, **p= 0.0033). Data were presented as mean ± SD of (C), (D), (F). The source data were provided in the Source data file. Lipid extraction, ultra-performance liquid chromatography, mass spectrometry, and lipid structural analyses were performed at Novo gene (Beijing, China) [48] . Bacterial cells (100 mg) were mixed with 0.75 mL methanol (#R40121, Thermo Fisher), which were vortexed in a glass tube with a Teflon lined cap. 2.5 mL of MTBE (#40477, Thermo Fisher) was added into the mixture and incubated for 1 h at room temperature in a shaker. Next, the upper (organic) phase was collected through centrifugation after adding 0.625 mL H 2 O. After that, 1 mL of the solvent mixture (MTBE/methanol/water (10:3:2.5, v/v/v)) was added into the lower phase to re-extract. Combined organicphases were dried and dissolved in 100 μL of isopropanol (#022906, Thermo Fisher) for storage. Then, the sample was detected by UHPLC-MS/MS using a Vanquish UHPLC system (Thermo Fisher, USA) coupled with an Orbitrap Q ExactiveTM HF mass spectrometer (Thermo Fisher, USA). Sample was injected into a Thermo Accucore C30 column (150 × 2.1 mm, 2.6 μm) using a 20 min linear gradient at a flow rate of 0.35 mL/min. The mobile phase buffer A was consisted of acetonitrile/water (6:4, v/v) with 10 mM ammonium acetate (#C21999, Thermo Fisher) and 0.1% formic acid (#LS118-4, Thermo Fisher), and buffer B was consisted of acetonitrile (#047138, Thermo Fisher)/isopropanol (#039194, Thermo Fisher) (1:9, v/v) with 10 mM ammonium acetate (#C21999, ThermoFisher) and 0.1% formic acid (#LS118-4, ThermoFisher). The solvent gradient was set as follows: 30% B, initial; 30% B, 2 min; 43% B, 5 min; 55% B, 5.1 min; 70% B, 11 min; 99% B, 16 min; 30% B, 18.1 min. Q ExactiveTM HF mass spectrometer was operated in positive [negative] polarity mode with sheath gas 40 psi, sweep gas 0 L/min, auxiliary gasrate 10 L/min [7 L/min], spray voltage 3.5 kV, capillary temperature 320 °C, heater temperature 350 °C, S-Lens RF level 50, scan range 114–1700 m / z , automatic gain control target 3e6, normalized collision energy 22 eV, 24 eV, 28 eV [22 eV, 24 eV, 28 eV], injection time 100 ms, isolation window 1 m / z , automatic gaincontrol target (MS2) 2e5, dynamic exclusion 6 s. The Compound Discoverer 3.01 (CD3.1, ThermoFisher) was used to perform peak alignment, peak picking, and quantitation of raw data for each metabolite. The peak intensities were normalized to the total spectral intensity base on these main parameters: retention time tolerance, 0.2 min; actual mass tolerance, 5 ppm; signal intensity tolerance, 30%; signal/noise ratio, 3; and minimum intensity, 100,000. Several databases were used for metabolite identification, including LipidBlast (( https://fiehnlab.ucdavis.edu/projects/LipidBlast ), Lipidmaps ( http://www.lipidmaps.org ) and Mtb LipidDB ( https://www.ncbi.nlm.nih.gov/pmc/articles/PMC3073466/ ). The mass error used was 5 ppm. Each sample was conducted in six independent replicates. Univariate analysis (t-test) was applied to calculate the statistical significance ( p value) and fold change of the metabolites between the means of the two groups using the statistical software R (version R-3.4.3), Python (version 2.7.6) and CentOS (CentOS release 6.6). Detection the levels of c-di-GMP in M. bovis BCG The yedH (mut)-overexpression ( yedH (mut)) and yedH -overexpression ( yedH ) of M. bovis BCG were constructed for detecting the levels of c-di-GMP. The c-di-GMP of M. bovis BCG strains were extracted using a modified protocol according to the following procedures [28] . 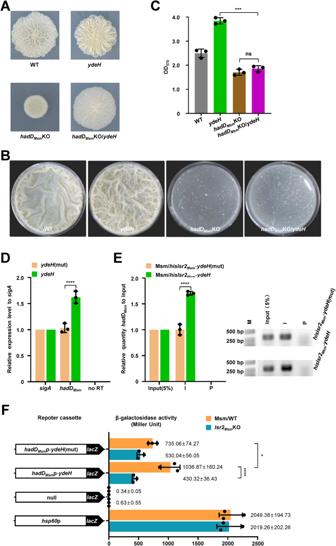Fig. 4: c-di-GMP promotes the expression ofhadDMsmby Lsr2Msmto affect biofilm formation inM. smegmatis. ASpot colony morphology of the wide type and itsydeH-overexpressed strains,hadDMsmknock-out and itsydeH-overexpression strains.BBiofilm formation of the WT,ydeH,hadDMsmKO, andhadDMsmKO/ydeHstrains.CQuantitation of biofilm biomass by crystal violet staining of the WT,ydeH,hadDMsmKO, andhadDMsmKO/ydeHstrains (n= 3, biological replicates). Two-tailed t-tests were performed for statistical analysis (***p= 0.0004).DRT-PCR quantitation ofhadDMsmtranscription in theydeH,ydeH(mut)-overexpressedM. smegmatisstrains. Two-tailed Student’s t-tests were performed for statistical analysis (****p< 0.0001). RT-PCR and gel analysis were performed under the same conditions and each experiment was performed three independent biological replicates. no RT was genomic DNA contamination control.EChIP assays for the effect of c-di-GMP on the intracellularhadDMsmp-binding activity of Lsr2MsminM. smegmatis. The input (5%) indicated that the supernatant of disrupted cells was diluted to 5%, ChIP using preimmune (P) or immune (I) sera raised against HisLsr2Msm. DNA of the input (5%), P, and I were used as temples for PCR (the right panel) (n= 3, biological replicates) and RT-qPCR (the light panel). M: DNA Marker. Two-tailed Student’s t-tests were performed for statistical analysis (****p< 0.0001).Fβ-galactosidase activity assays. The effect of c-di-GMP on Lsr2Msmregulates the expression ofhadDMsmwas assayed by overexpressing pMV261-hadDMsmp-ydeH-lacZand pMV261-hadDMsmp-ydeH(mut)-lacZplasmids in the Msm/WT,lsr2MsmKO strains (n= 3, biological replicates). None promoter-lacZandhsp60p-lacZplasmids overexpression were used as controls. Two-tailed Student’s t-tests were performed for statistical analysis (*p= 0.0414, ****p< 0.0001). Data were presented as mean ± SD of (C), (D), (E), (F). The source data were provided in the Source data file. 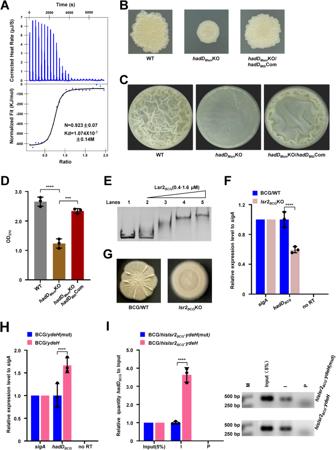Fig. 5: The c-di-GMP signal regulatory system is conserved in mycobacteria includingM. tuberculosis. AITC assays for the interaction between Lsr2Mtband c-di-GMP. Original titration data and integrated heat measurements are shown in the upper and lower plots.BSpot colony morphology of the wide type,hadDMsmknock-out andhadDMtbcomplementary strains.CBiofilm formation of the WT,hadDMsmKO, andhadDMtbcomplementary strains.DQuantitation of biofilm biomass of the WT,hadDMsmKO, andhadDMtbcomplementary strains by crystal violet staining (n= 3, biological replicates). Two-tailed t-tests were performed for statistical analysis (****p< 0.0001, ***p= 0.0004).EEMSA assays for the effect of c-di-GMP onhadDBCGpromoter DNA-binding activity of Lsr2BCG.hadDBCGp was co-incubated with increasing concentration of Lsr2BCG(lanes 2–5). Three independent experiments were performed.FRT-PCR for transcriptional analysis ofhadDBCGin the WT,lsr2BCGKOM. bovisBCG strains (n= 3, biological replicates). Two-tailed Student’s t-tests were performed for statistical analysis (****p< 0.0001). RT-PCR and gel analysis were performed under the same conditions.GSpot colony morphology of the WT andlsr2BCGknock-out BCG strains on 7H10 plates.HRT-PCR for transcriptional analysis ofhadDBCGin theydeH(mut),ydeH-overexpressedM. bovisBCG strains (n= 3, biological replicates). Two-tailed Student’s t-tests were performed for statistical analysis (****p< 0.0001).IChIP assays for the effect of c-di-GMP on the intracellular DNA-binding activity of Lsr2BCGin theM. bovisBCG strains. The input (5%) indicated that the supernatant of disrupted cells was diluted to 5%, ChIP using preimmune (P) or immune (I) sera raised against HisLsr2BCG. DNA sample of the input (5%), P, and I were used as temples for PCR (the right panel) (n= 3, biological replicates) and were quantified using RT-qPCR (the light panel). M: DNA marker. Two-tailed Student’s t-tests were performed to for statistical analysis (****p< 0.0001). Data of figures (D), (F), (H), and (I) were presented as mean ± SD. The source data were provided in the Source data file. 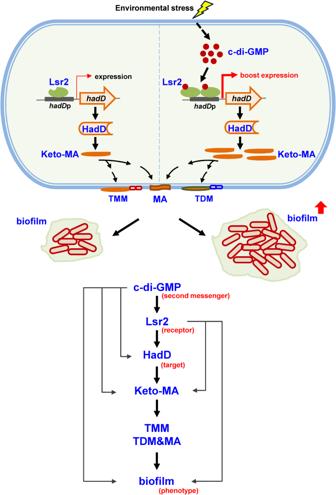Fig. 6 The model of which c-di-GMP stimulates the expression ofhadDby Lsr2 to control biofilm formation in mycobacteria. The strains were cultured to an OD 600 = 1.2, and cells were collected and washed twice with PBS buffer. Subsequently, cells were suspended in 15 mL ddH 2 O and crushed using ultrasound at 450 W for 1 h. The samples were centrifuged. Then, the supernatant was extracted with phenol/chloroform and concentrated to 1.5 mL. Finally, the levels of c-di-GMP were quantified using an ELISA kit (#F20205-B, FANKEWEI). Reporting summary Further information on research design is available in the Nature Portfolio Reporting Summary linked to this article.